Global pattern for the effect of climate and land cover on water yield Research results on the effects of land cover change on water resources vary greatly and the topic remains controversial. Here we use published data worldwide to examine the validity of Fuh’s equation, which relates annual water yield ( R ) to a wetness index (precipitation/potential evapotranspiration; P / PET ) and watershed characteristics ( m ). We identify two critical values at P / PET =1 and m =2. m plays a more important role than P / PET when m <2, and a lesser role when m >2. When P / PET <1, the relative water yield ( R / P ) is more responsive to changes in m than it is when P / PET >1, suggesting that any land cover changes in non-humid regions ( P / PET <1) or in watersheds of low water retention capacity ( m <2) can lead to greater hydrological responses. m significantly correlates with forest coverage, watershed slope and watershed area. This global pattern has far-reaching significance in studying and managing hydrological responses to land cover and climate changes. The effects of land cover changes on water resources have been debated for many years. Numerous studies have been conducted throughout the world to address this concern. The paired-watershed experiment (PWE) method [1] , which is believed to accurately quantify the change in water yield caused by vegetation changes, has been widely used in the past century [2] , [3] . Several reviews of these experiences involving more than 250 PWEs from around the globe have reported that, although forest changes significantly affect the water yield [3] , [4] , [5] , the magnitude of any change varies greatly from one watershed to another [6] , [7] . Some studies, especially in large watersheds, found that forest changes have limited effects [8] , no effects [9] , [10] or even positive effects [11] , [12] on water yield. These highly variable and apparently inconsistent results have led to debates in both research and resource management communities, especially when another catastrophic flood or drought occurs somewhere in the world [13] . Clearly, a unifying theory describing the influence of climate and land cover on water yield, and which is validated by global experimental studies, would improve our understanding on the underlying mechanisms and support natural resource management. Along with ‘bottom-up’ experimental approaches, energy-based theoretical equations describing climate and water balance have been developed and applied in what is often called a top-down approach [14] , [15] , [16] . Among them, frameworks by Budyko [17] and Fuh [18] have received the most attention and application [19] . Both frameworks consider climate as well as a watershed-specific parameter. Recently, the two frameworks were shown to be virtually identical [20] , with the Fuh’s equation being a more generalized form [19] . However, neither framework has been comprehensively analysed using a global data set nor have possible mechanisms to explain emerging patterns been offered. A universal model that incorporates precipitation ( P ), potential evapotranspiration ( PET ) and watershed characteristics to explain the variable hydrological responses to land cover changes is needed. In this study, a theoretical pattern on the dependence of the ratio of annual water yield to precipitation on wetness index ( P / PET ) and watershed characteristics ( m ) based on Fuh’s equation [18] is analysed and validated using the globally published data. We confirm that the Fuh’s theoretical equation is a valid and useful framework for studying land cover changes and hydrological responses. Theoretical analyses identify two critical values at P / PET =1 and m =2. P / PET plays a more important role than m when m >2, and less when m <2. When P / PET <1, the sensitivities of R / P to m values are more dramatic and multi-directional than those when P / PET >1, suggesting that any land cover changes in non-humid regions ( P / PET <1) can lead to greater and more sensitive hydrological responses. Relative contributions of P / PET and m to annual water yield at a large spatial scale are mapped out globally. The m values are significantly correlated with forest coverage or treated area in PWE, watershed area and slope. The pattern explains the great variability in the effect of forest cover changes on water yield and implies that the effect can be negative, neutral or even positive, depending on the P / PET and m values of a watershed. Performance and validation of the pattern Equation (1) depicts the dependence of the ratio ( R / P ) of annual water yield ( R ) to precipitation ( P ) on P and PET (see Methods): where R / P is a dimensionless annual water yield coefficient; P / PET is a dimensionless variable often called wetness index that differs by region and year, with its reciprocal ( PET / P ) often called dryness index; and m (1, ∞) is an integration constant that is dimensionless and independent of P and PET , and represents watershed characteristic [18] , [21] . One extreme case occurs when m =1, R / P =1, where all precipitation becomes streamflow and residence time is 0. The opposite extreme case occurs when m →infinity, R / P =0 ( PET > P ) or R / P =1−( P / PET ) −1 ( PET < P ), where all precipitation remains in the watershed and residence time equals the time for all precipitation to evaporate. Thus, m indicates the ability for a watershed to retain water for evapotranspiration; larger m values mean larger and longer water retention capacities. The variable m can be used to denote watershed characteristics, including watershed area, slope, land cover and other characteristics (for example, soil texture, depth). From the equation (1), the sensitivity functions of R / P to P / PET and m are given as: The results of equations (1)–(3), ,  are illustrated in Fig. 1 . 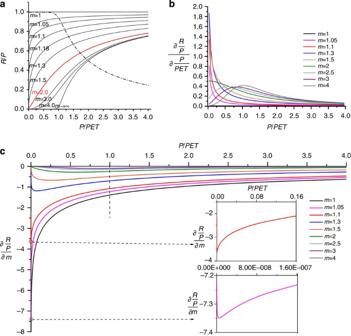Figure 1: Theoretical distributions of the pattern and two sensitivity functions. (a) Distribution of the pattern, red line is the curvem(watershed characteristics)=2 and dashed line is the curve of maximum ΔR/P(difference inR/P(water yield coefficient) betweenm=1 andm=∞) withP/PET(wetness index). (b) Distribution of the sensitivity function ofR/PtoP/PET, green line is the curvem=2; when 1<m≤2,decreases rapidly and monotonically withP/PET, while whenm>2changes withP/PETin unimodal curves. (c) Distribution of the sensitivity function ofR/Ptom, dashed line isP/PET=1, the two small panels showing finer scale ofP/PET; when 0<P/PET≤1,changes withP/PETdramatically with multiple directions, while whenP/PET>1changes smoothly and monotonically withP/PET. Figure 1: Theoretical distributions of the pattern and two sensitivity functions. ( a ) Distribution of the pattern, red line is the curve m (watershed characteristics)=2 and dashed line is the curve of maximum Δ R / P (difference in R / P (water yield coefficient) between m =1 and m =∞) with P / PET (wetness index). ( b ) Distribution of the sensitivity function of R/P to P/PET , green line is the curve m =2; when 1< m ≤2, decreases rapidly and monotonically with P / PET , while when m >2 changes with P / PET in unimodal curves. ( c ) Distribution of the sensitivity function of R/P to m , dashed line is P / PET =1, the two small panels showing finer scale of P / PET ; when 0< P / PET ≤1, changes with P / PET dramatically with multiple directions, while when P / PET >1 changes smoothly and monotonically with P / PET . Full size image According to equation (1), R/P changes with P / PET and m within the theoretical range defined by the five boundaries of P / PET =0, P / PET =∞, R / P =1 ( m =1), R / P =0 ( P / PET <1 and m →∞) and R / P =1−( P/ PET ) −1 ( P / PET >1 and m →∞), which are shown in Fig. 1a . We verified equation (1) with the globally published data ( Supplementary Data 1 for time-trend studies and Supplementary Data 2 for PWE studies. The time-trend studies are defined as those that provide circumstantial evidence of the influence of watershed management on water yield [3] ). First, this hypothetical universal pattern captured the majority of the data regarding the changes in R / P with P / PET for four land cover types (forest, shrub, grass/crop and mixed lands). More than 90% of the data on R / P with P / PET , as shown in Fig. 2a and listed in Supplementary Data 1 , and more than 88% of the data on R / P with P / PET , as shown in Fig. 2b and listed in Supplementary Data 2 , fit within the theoretical range. Second, the curves in Fig. 2a,b are all statistically significant ( p <0.001). The one-way analysis of variance shows that the differences in m values between any two of the four land cover types and between the forested and non-forested watersheds were all significant ( p <0.001). This suggests that land cover changes significantly modify m values, and an increase in forest coverage indeed reduces R / P , which is consistent with the general conclusions from PWE studies [3] , [5] , [13] . 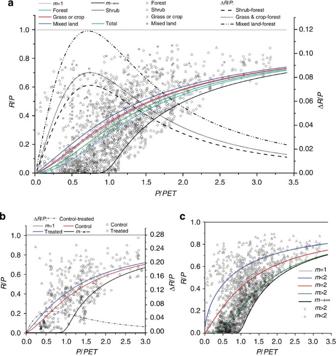Figure 2: Validation of the pattern using global observed water yield coefficient. (a) Ninety percent ofSupplementary Data 1fall within the theoretical range; the five coloured lines: forest (n=1,187,m=2.83,p<0.001), shrub (n=271,m=2.33,p<0.001), grassland or cropland (n=233,m=2.28,p<0.001), mixed land (n=237,m=2.12,p<0.001) and the total (n=1,928,m=2.54,p<0.001); the three dashed lines are the ΔR/Ps (differences inR/P(water yield coefficient) between forest and the other three respective land covers). (b) Eighty-eight percent ofSupplementary Data 2fall within the theoretical range; the two coloured lines: forested (n=234,m=2.32,p<0.001) and non-forested (n=234,m=2.05,p<0.001); the dashed line is the ΔR/P(difference inR/Pbetween forested and non-forested). (c) The critical valuem(watershed characteristics)=2 (red line) dividing the changes ofR/PwithP/PET(wetness index) into two apparently different patterns (m<2 (blue line) andm>2 (green line)). Figure 2: Validation of the pattern using global observed water yield coefficient. ( a ) Ninety percent of Supplementary Data 1 fall within the theoretical range; the five coloured lines: forest ( n =1,187, m =2.83, p <0.001), shrub ( n =271, m =2.33, p <0.001), grassland or cropland ( n =233, m =2.28, p <0.001), mixed land ( n =237, m =2.12, p <0.001) and the total ( n =1,928, m =2.54, p <0.001); the three dashed lines are the Δ R / P s (differences in R / P (water yield coefficient) between forest and the other three respective land covers). ( b ) Eighty-eight percent of Supplementary Data 2 fall within the theoretical range; the two coloured lines: forested ( n =234, m =2.32, p <0.001) and non-forested ( n =234, m =2.05, p <0.001); the dashed line is the Δ R / P (difference in R / P between forested and non-forested). ( c ) The critical value m (watershed characteristics)=2 (red line) dividing the changes of R / P with P / PET (wetness index) into two apparently different patterns ( m <2 (blue line) and m >2 (green line)). Full size image Theoretically, R / P increases with P / PET for all m (1, ∞) and decreases with m for all P / PET (0, ∞) ( Fig. 1a ). Correspondingly, the sensitivities of R / P to P / PET are above 0 ( Fig. 1b ), while these to m are below 0 ( Fig. 1c ). Our theoretical analysis from equations (1)–(3), ,  identified two critical values m =2 and P / PET =1 (see Methods). When 1< m ≤2, decreases rapidly and monotonically with increasing P / PET . In contrast, when m >2, changes with P / PET as unimodal curves ( Fig. 1b ), with the P / PET values of inflection points increasing with m from the starting point m =2 and P / PET =0. The critical value of m =2 is also supported by the published data as shown in Fig. 2c where there are two different patterns of R / P in response to P / PET for m <2 and m >2. Thus, our theoretical analyses and global data indicate that hydrological responses to land cover changes are more sensitive when watersheds have lower water retention capacity (1< m <2), probably due to the dominance of low water retention land types (for example, open or sparsely vegetated natural land cover types or disturbed land cover types) or other watershed characteristics of low water retention capacity (for example, small watershed area, thin soils, shallow bedrocks, low infiltration capacities, steep watershed slopes). The sensitivity of R / P to m varies with P / PET in unimodal curves for all m values (1, ∞), but they are not symmetrical to P / PET ( Fig. 1c ). When P / PET >1, the absolute values of decrease smoothly and monotonically with P / PET for all m values (1, ∞). In extremely wet environments ( P / PET >>1), hydrological responses are neither sensitive to m nor sensitive to P / PET ( Fig. 1c ). When 0< P / PET ≤1, the absolute values of change with P / PET in unimodal curves for all m values (1, ∞), with the P / PET values of inflection points increasing monotonically from 0 to 1 when m changes from 1 to ∞. For any given m value, the highest sensitivity of R / P to m occurs at 0< P / PET <1. In extremely dry environments ( P / PET ≪ 1), the smaller the m is, the greater the sensitivity of R / P to m and P / PET will be, and vice versa ( Fig. 1c ). Theoretically, all Δ R / P values between any two different m values, including the maximum Δ R / P between m =1 and m =∞, change with P / PET in unimodal curves with the peak values falling in the P / PET range of 0 to 1 ( Fig. 1a ). Clearly, the P / PET values of inflection points lie between 0 and 1 with their actual values varied by m . The global data set shows that Δ R / P values between forest cover and any one of the other three land covers in the time-trend studies (with m values ranging from 2.12 to 2.83 as shown in Fig. 2a ) and between the forested and non-forested types of PWE studies (with m values ranging from 2.05 to 2.32 as shown in Fig. 2b ) change with P / PET as unimodal curves with their peak values at the P / PET values of 0.5–0.7 ( Fig. 2a,b ), which are within the theoretical P / PET range of (0, 1). In addition, much higher coefficients of variation (CV) in the globally published R / P also fall in the P / PET range of (0, 1) ( Fig. 3 ). Thus, any land cover changes in the regions with P / PET <1 (non-humid regions) can potentially cause higher and more sensitive impacts on water yields. 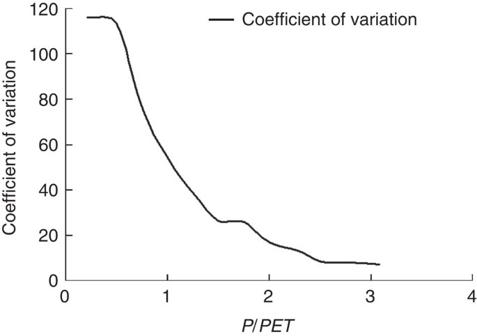Figure 3: Changes in coefficient of variation of globally observed water yield coefficient with wetness index. For all the gathered data in Supplementary Data 1, we calculated theCV(coefficient of variation) in every sub-range (0–0.2, 0.2–0.4, 0.4–0.6…,) ofP/PET(wetness index) according toCVi=Si/Xi(CViis theCVof the sub-range;Siis the standard deviation;Xiis the mean value) (see Methods). Figure 3: Changes in coefficient of variation of globally observed water yield coefficient with wetness index. For all the gathered data in Supplementary Data 1, we calculated the CV (coefficient of variation) in every sub-range (0–0.2, 0.2–0.4, 0.4–0.6…,) of P/PET (wetness index) according to CV i = S i / X i ( CV i is the CV of the sub-range; S i is the standard deviation; X i is the mean value) (see Methods). Full size image In summary, we conclude that equation (1) and its derived equations (2) and (3) are a robust framework for studying global land cover patterns and water yields, and two critical values ( m =2 and P / PET =1) exist for defining hydrological sensitivities. The factors influencing m and changed water yield in PWEs We further related the m values to various watershed variables given in Supplementary Data 1 and 2 . The m values were positively related to forest coverage (or treated forested area for the PWE studies; p <0.001) and watershed area ( p <0.001) and negatively to watershed slope ( p <0.001). In addition, we related the change in water yield coefficient (Δ R / P ) to the land cover changes, watershed area and watershed slope for the PWE studies. While Δ R / P increased significantly with treated area percentages ( Fig. 4a ) as previously reported [3] , Δ R / P also increased ( p <0.001) with watershed slope ( Fig. 4b ) but decreased ( p <0.001) with watershed area ( Fig. 4c ). Thus, R / P is not only affected by P / PET , but also by changes in land cover and difference in the watershed parameter, which highlights the fact that the effects of land cover changes on water yield are influenced by watershed characteristics and thus are watershed specific [22] . 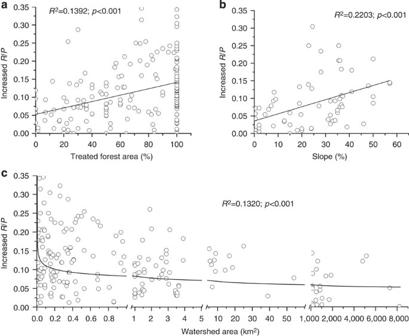Figure 4: Relationships of the change in water yield coefficient with various factors in PWE. (a) Relationship with the percentage of treated area (n=181,p<0.001); (b) relationship with the watershed slope (n=70,p<0.001); (c) relationship with the watershed area (n=214,p<0.001). Figure 4: Relationships of the change in water yield coefficient with various factors in PWE. ( a ) Relationship with the percentage of treated area ( n =181, p <0.001); ( b ) relationship with the watershed slope ( n =70, p <0.001); ( c ) relationship with the watershed area ( n =214, p <0.001). Full size image Relative contributions of P / PET and m to R / P The global distributions of P / PET and m values are shown in Fig. 5 (see Methods). Percentages of the global areas with P / PET <1 and m >2 are 68.9 and 74.1%, respectively. 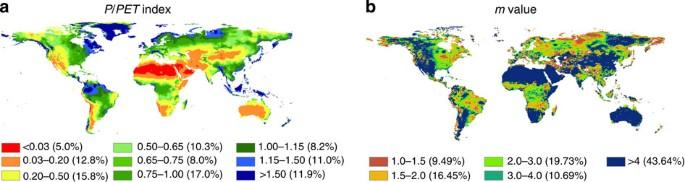Figure 5: Global distributions of wetness index and watershed characteristic values. (a)P/PET(wetness index) values; (b)m(watershed characteristics) values. Figure 5: Global distributions of wetness index and watershed characteristic values. ( a ) P / PET (wetness index) values; ( b ) m (watershed characteristics) values. Full size image To quantify the relative roles of P / PET and m in R / P , we estimated their relative contributions, C P / PET and C m , respectively ( Fig. 6 ). When m >2, P / PET has a larger role in R / P than m , while when m <2, m becomes more important. This theoretical result is congruent with the global published data where the averaged relative contributions of m are 72 and 15% for 1< m <2 and m >2, respectively, with 28 and 85% for their corresponding P / PET values. 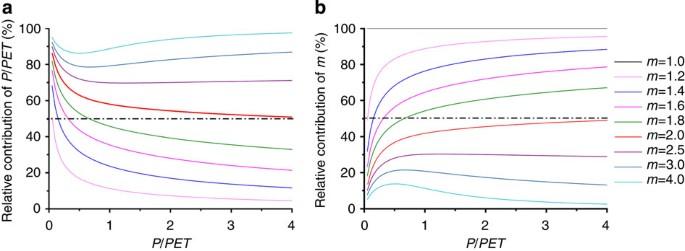Figure 6: Relative contributions of wetness index and watershed characteristics to water yield coefficient. (a) Relative contributions ofP/PET(wetness index) toR/P(water yield coefficient); (b) relative contributions ofm(watershed characteristics) toR/P. Figure 6: Relative contributions of wetness index and watershed characteristics to water yield coefficient. ( a ) Relative contributions of P / PET (wetness index) to R / P (water yield coefficient); ( b ) relative contributions of m (watershed characteristics) to R / P . Full size image On the basis of the distributions of P / PET and m values shown in Fig. 5 , the worldwide C P / PET and C m in percentages as well as the patterns of m -dominated and P / PET -dominated zones are mapped in Fig. 7 . The P / PET -dominated zones ( C P / PET >60% or C m <40%) amount to 70.4%, while m -dominated zones ( C m >60% or C P / PET <40%) are 13.8%, and the rest are 15.8% where both P / PET and m have a similar role in runoff. This result is consistent with the case study in Murray–Darling basin, Australia [19] , where the C P / PET and C m , according to Fig. 6 , are 75.4 and 24.6%, respectively, with its m being 2.465 and P / PET being 0.287. The two percentages are close to our corresponding values of 76.1 and 23.9% in Fig. 7a . In addition, the result from Fig. 7a is strongly supported by the data in Supplementary Data 1 , as there were significant correlations between them ( n =19, R 2 =0.74, p <0.001 for large watersheds (>2,500 km 2 comparable to 0.5° (lat.) × 0.5° (long.) grid pixel) and n =125, R 2 =0.085, p <0.001 for all watersheds). 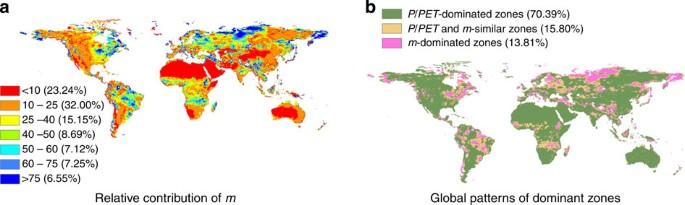Figure 7: Global patterns for the contributions of wetness index and watershed characteristics to water yield coefficient. (a) Relative contributions ofm(watershed characteristics) orP/PET(wetness index) toR/P(water yield coefficient); (b) global patterns ofm- andP/PET-dominated zones (P/PET-dominated zones:Cm<40% orCP/PET>60%;P/PETandm-equal zone:CmorCP/PET=40–60%;m-dominated zones:Cm>60% orCP/PET<40%;CmandCP/PETare the relative contributions ofmandP/PET, respectively;CP/PET=100−Cm). Figure 7: Global patterns for the contributions of wetness index and watershed characteristics to water yield coefficient. ( a ) Relative contributions of m (watershed characteristics) or P / PET (wetness index) to R / P (water yield coefficient); ( b ) global patterns of m - and P / PET -dominated zones ( P / PET -dominated zones: C m <40% or C P / PET >60%; P / PET and m -equal zone: C m or C P / PET =40–60%; m -dominated zones: C m >60% or C P / PET <40%; C m and C P / PET are the relative contributions of m and P / PET , respectively; C P / PET =100− C m ). Full size image Using the globally published data, this study confirms that equation (1) derived from Fuh’s equation is a valid framework for the effects of climate and land cover on hydrology. More importantly, we clarified the relative roles of climate and watershed characteristics on hydrological response. When interpreting various Budyko-based coupled curves or equations [2] , [14] , [20] , [23] , the common perception is that hydrological responses are mainly driven by precipitation (climate) and PET (energy) with the watershed parameter playing a secondary role [14] , [24] . However, the relative contributions of the watershed parameter and climate to hydrological responses have never been fully examined and quantified. Without those quantifications, the above perception is questionable. Our theoretical analysis shows that m can play a more important role in hydrological responses than P / PET when m <2, while m plays a lesser role when m >2. This result is supported by empirical analysis of the globally published data where the averaged relative contributions of m are 72 and 15% for 1< m <2 and m >2, respectively. Clearly, both our theoretical and empirical analyses demonstrate that the role of m can be larger than P / PET in hydrological responses, even though P / PET plays a dominant role in most of the regions of the world. This conclusion is different from the commonly held perception that climate plays the dominant role and watershed characteristics ( m ) are secondary. The critical value of m =2 defines the high (1< m <2) and low ( m >2) sensitivity ranges for hydrological response ( R / P ) to changes in m . Zhang et al. [14] also noted the different hydrological responses with respect to various values of the watershed parameter, but failed to find the critical value. When m >2, the water retention capacity in a watershed is high, probably due to the combination of high vegetation cover, mixed forest type [25] , large watershed area, gentle slopes and high soil infiltration capacity. In this case, the hydrological effects of any land cover change in m (for example, deforestation, urbanization) will likely be buffered. In contrast, when m <2, the water retention capacity in a watershed is low, probably due to the combination of poorer vegetation cover, simplified forest type [25] , small watershed area, steeper slopes and lower soil infiltration capacity. Under this situation, the hydrological responses are more sensitive to any land cover-induced change in m . The large role of m in hydrological responses is supported by published studies [26] , [27] , [28] , which shows that land cover change can significantly alter m values and lead to a larger role in hydrological responses than climate ( P / PET ). Climatic variability and land cover/land-use changes are commonly recognized as two major drivers for hydrological variations, and consequently their strengths, directions and interactions control future water supply and flow regimes. Unfortunately, current climate change impact studies predict future water supply based only on various climate change scenarios without specific consideration of land cover or land-use changes, which may either underestimate or overestimate the impacts of climate change on water resources. In contrast, the majority of PWE studies exclude the impacts of climatic variability so that the impacts of forest changes on hydrology can be determined. This approach may not provide a full picture on how climate and forest change interactively affect hydrology. Therefore, inclusion of both m and P / PET in future water resource assessment is critical for understanding and managing water resources. Our results show that annual water yield is more sensitive to land cover change ( m ) in water-limited regions ( P / PET <1), as indicated by higher CV, non-symmetrical shapes and multiple changing directions in R / P , as compared with those when P / PET >1 ( Figs 1b,c and 3 ). In water-limited environments ( P / PET <1), forests normally develop deeper and larger root systems to access more soil water. This strategy allows forests to survive. Conversely, any changes to forests (for example, deforestation or conversion to other land-use types) can lead to larger hydrological responses (for example, larger water yields). The above conclusion is supported by various case studies. For example, the relative contribution of m to R / P in the Yellow River basin, China, was estimated as 89.1% (ref. 29 ), which is much higher than that estimated 41.9% response in the Miramichi River basin in Canada [30] , when their P / PET were markedly different (0.51 and 1.91, respectively) and their m values were similar (1.51 and 1.40, respectively). Another useful comparison is that between Manuel Diaz basin in Uruguay [31] and Lookout Creek watershed, near Eugene, Oregon, USA [32] where their relative contributions were 86.9 and 34.1%, when their P / PET were markedly different (0.95 and 2.91, respectively) and their m values were similar (1.68 and 1.53, respectively). Zhang et al. [14] showed that E / P is most sensitive to changes in watershed characteristics for the regions with the dryness index ( PET / P ) around 1. However, our theoretical analysis ( Fig. 1c ) showed that the greatest sensitivities fall in the regions of P / PET <1, the P / PET value at which the greatest sensitivity of R / P to m is reached increases from 0 to 1 with m changing from 1 to ∞. Our analysis from the globally published data ( Fig. 2a,b ) also shows that the P / PET values of maximum Δ R / P fall in the range of 0.5–0.7 for the averaged m values varying from 2.05 to 2.83. According to our framework, the water yield coefficient ( R / P ) is determined by just three variables ( P , PET and m ) or even two independent ones ( P / PET and m ). Using the globally published data from time-trend studies and PWE studies, this paper shows that the m values and change in water yield coefficient (Δ R / P ) are significantly correlated with proportion of forest coverage, watershed area and slope, although each coefficient of determination is relatively low. The reason for the low coefficients of determination may be that m or Δ R / P is influenced by many factors and thus the contribution of each single factor is small. In this study, we identified three key variables influencing m values and Δ R / P based on the limited data we have. It is likely that many other variables may also contribute to water yields [33] , [34] , [35] , [36] . Nevertheless, the significant relationship between m and the three identified key variables indicated that any changes in those variables can alter m values and consequently lead to changes in Δ R / P . Deforestation may decrease water retention ability or m values and thus increase water yield due to accelerating water movement as a result of fewer obstacles and surface soil compaction [37] . In contrast, reforestation may increase water retention ability or m values and thus decrease water yield through decelerating water movement as a result of more obstacles, longer flow paths and poriferous surface soils. With respect to slope, the watersheds with steeper slopes normally have lower water retention ability or smaller m values and thus higher water yields due to its faster water movement and consequently shorter residence time of liquid water. Watershed area can be an important variable for hydrological responses. Compared with small-sized watersheds, large ones tend to have higher water retention capacities (greater m values) and consequently lower hydrological responses mainly due to their more complex landforms (for example, lakes, wetlands), greater buffering capacities and longer residence times. Changes in forest cover have been shown to influence water yield in small watersheds, but it is unclear if this result holds for large basins [38] . Researchers have showed that forest changes in large watersheds have limited effects [8] , no effects [9] , [10] or even positive effects [11] , [12] on water yield. The inconsistency may be explained through our framework. Compared with small watersheds, large ones usually have higher m values due to greater areas and gentler slopes [8] . Thus, it is expected that the same forest changes in large watersheds will cause less change in m values, with the result that there is less effect on water yield than in small watersheds. If m values of some large watersheds are much higher than two ( m >>2), forest changes will have no effects on water yield. In humid regions ( P / PET >1) where PET plays a dominant role in water yield or evapotranspiration, a decrease in PET will likely cause a significant increase in water yield. This is consistent with the findings that afforestation can increase water yield in large watersheds of humid regions [11] , [12] because afforestation cools local land surface temperature [39] and thus decreases PET . Our results on the unifying framework and the relationship between m and watershed characteristics have far-reaching implications for scientific research and natural resource management. First, the verified Fuh’s equation can be used as a top-down framework for studying and managing the effects of climate and land cover changes on water resources. It also opens up new research opportunities for studying how climate and watershed characteristics interactively affect hydrology, and what hydrological responses might occur under specific m and P / PET values. Second, we have clarified and quantified the relative roles of climate and watershed characteristics in hydrological response and challenged the commonly held perception that climate plays a dominant role while watershed characteristic is secondary. Correctly understanding the relative roles and possible interactions of watershed condition ( m ) and climate ( P / PET ) in hydrological response is crucial for predicting and managing future water resources and their associated ecological services under climate and land cover changes. Third, the critical values ( m =2 and P / PET =1) we identified can provide important guides for determining hydrological sensitivities to any changes in climate and land cover. Specifically, the most sensitive regions in the world are those where m is <2 and P / PET <1. Finally, large variations in hydrological response suggest that any extrapolation of research results from one watershed to others must be done with caution. This study has made incremental advancement on several important aspects of the energy framework (namely, Budyko and Fuh’s equations or curves), but like all studies there are some uncertainties in this research. The uncertainties come from several sources. First, the global published data used in this study are from various case studies where different methods (for example, PWE, time-trend studies) are applied, which may cause a level of uncertainty in our data. Second, the time period over which the data were collected may not include all representative responses of water yields to P / PET and m . Third, the data are mainly from the regions where the research is concentrated because of management concerns, suggesting that our data set may not well cover the regions where there are no or less management interests or concerns (for example, extremely arid areas). Each of these aspects may create uncertainties, which calls for the need for both empirical and modelling studies using comparable methods in all representative parts of the world. Derivation of equation (1) Fuh’s model [18] can be written as: where E is evapotranspiration from a watershed and the other variables have the same meanings as those in equation (1). Both P / PET and PET / P have been used as the surrogate of climate in various water–energy equations [2] , [23] , [40] , [41] . In this study, we used P / PET instead of PET / P as the former offers several important advantages. First, PET is always larger than 0 and relatively stable in a given region as it is determined by available energy. In contrast, P may be 0 in some extremely arid areas (for example, deserts), which can lead to infinite values of PET / P. Therefore, P / PET falls in clearly defined and limited boundary ranges in any given region (for example, 0–4 in our study), while PET / P may have infinite boundary ranges (for example, from 0.25 to infinite in our study) that make analysis more difficult. Second, because of the difference in the boundary ranges, using P / PET allows more effective quantifications on the hydrological sensitivity of R / P to P / PET than using PET / P , especially for the areas with P / PET <1 in which R / P is more sensitive to P / PET and m values. The general water balance equation for a watershed can be written as: where R is total water yield including surface runoff, interflow and baseflow and Δ W is change of watershed water storage. For a whole water year, Δ W ≈0, there will be equation (6): Equation (1) can be derived by substituting E in equation (6) with equation (4). Estimation of yearly PET Yearly PET was estimated using Hamon’s method [42] , [43] . where D is the time from sunrise to sunset in multiples of 12 h, varies with date, latitude, slope and aspect of a watershed (if the influences of slope and aspect are not considered, the average daily D of an entire year is 1). V d is the saturated vapour density (g m −3 ) at the annual mean temperature ( T , °C), V d =216.7 × V s /( T +273.3); V s is the saturated vapour pressure (mb), V s =6.108 × exp[17.26939 × T/ ( T +237.3)]. K is the correction coefficient to adjust PET calculated using Hamon’s method to realistic values. Comparing the reported PET s with the calculated PET s for some PWE and time-trend studies, we found that the K values to adjust the two types of PET s ranged from 1.2 to 1.4. Thus, to keep consistency, we used K =1.3 to calculate the PET s of all PWE and time-trend studies in Supplementary Data 1 and 2 , even for those studies that had PET s reported. Determination of the two critical values P / PET =1 and m =2 The second derivatives of equation (1) or the first derivatives of equations (2) and (3) are given as follows: is above 0 for all P / PET (0, ∞) and m (1, ∞) values, showing that the is increasing with m (1, ∞). When m <2, is below 0 for all P / PET (0, ∞), showing that the is decreasing with P / PET (0, ∞). When m =2, at P / PET →0. When m >2, for any given m value (2, ∞), there is an inflection point at which the changes with P / PET from above 0 to below 0, and correspondingly, changes with P / PET from uptrend to downtrend. A mathematical theorem guarantees the correctness of the claim . We have also demonstrated the conclusion through respective derivatives. When P / PET >1, is above 0 for all m (1, ∞), showing that the is increasing with P / PET (1, ∞). When P / PET =1, at m →∞. When P / PET <1, for any given m value (1, ∞), there is an inflection point at which the changes with P / PET from below 0 to above 0, and correspondingly, changes with P / PET (0,1) from downtrend to uptrend. We summarized the above analyses in Table 1 . Table 1 Changes of the two sensitivity functions with wetness index and watershed characteristics. Full size table CV of globally published R / P data For all the gathered data in Supplementary Data 1 , we calculated the CV in every sub-range (0–0.2, 0.2–0.4, 0.4–0.6,…) of P / PET according to (CV i is the CV of the sub-range; S i is the standard deviation; is the mean value). The relative contributions of P / PET ( C P / PET ) and m ( C m ) On the basis of equations (2) and (3), we calculated the ratio ( α ) of . C P / PET and C m were calculated according to: Global distributions for various parameters Using data on global annual runoff ( R ) and precipitation ( P ) ( http://www.sage.wisc.edu/atlas/maps.php?datasetid=41&includerelatedlinks=1&dataset=41 ) and PET ( http://www.cgiar-csi.org/data/global-aridity-and-PET-database ), we calculated the global P / PET and hence estimated global m values according to equation (1). The estimated global m values and global wetness index ( P / PET ) were then used as inputs to equations (2) and (3) to calculate the global sensitivities of R / P to P / PET and m . Finally, the global sensitivities of R / P to P / PET and m were used to calculate the relative contributions of P / PET and m to R / P according to equations (13) and (14). All the above results were integrated to develop the world maps at the grid size of 0.5° (latitude) × 0.5° (longitude). Statistic analysis Correlations between any two parameters are calculated using OriginLab OriginPro 9.0.0. All recorded forest coverage (or treated forest area), watershed slope and watershed area in Supplementary Data 1 and 2 are used to calculate the relationship between m values (or Δ R / P ) and any one of the watershed characteristics. The C m for large watersheds (>2,500 km 2 ) in Supplementary Data 1 and 2 were directly related to the C m in Fig. 7a . However, the C m for smaller watersheds were averaged in each pixel (2,500 km 2 ) and then related to the C m in Fig. 7a . How to cite this article : Zhou, G. et al. Global pattern for the effect of climate and land cover on water yield. Nat. Commun. 6:5918 doi: 10.1038/ncomms6918 (2015).